Mutations in filamin C cause a new form of familial hypertrophic cardiomyopathy Mutations in different genes encoding sarcomeric proteins are responsible for 50–60% of familial cases of hypertrophic cardiomyopathy (HCM); however, the genetic alterations causing the disease in one-third of patients are currently unknown. Here we describe a case with familial HCM of unknown cause. Whole-exome sequencing reveals a variant in the gene encoding the sarcomeric protein filamin C (p.A1539T) that segregates with the disease in this family. Sequencing of 92 HCM cases identifies seven additional variants segregating with the disease in eight families. Patients with FLNC mutations show marked sarcomeric abnormalities in cardiac muscle, and functional analysis reveals that expression of these FLNC variants resulted in the formation of large filamin C aggregates. Clinical studies indicate that FLNC -mutated patients have higher incidence of sudden cardiac death. On the basis of these findings, we conclude that mutations in the gene encoding the sarcomeric protein filamin C cause a new form of familial HMC. Hypertrophic cardiomyopathy (HCM) is a relatively frequent and potentially devastating disease, which affects 1:500 individuals and represents one of the main causes of sudden cardiac death among young adults [1] , [2] . The study of familial HCM cases has revealed that mutations in at least 11 different genes encoding sarcomeric proteins are responsible for 50–60% of these familial cases [3] , [4] . However, in about one-third of patients with a family history of HCM, the genetic alterations causing the disease are currently unknown, and this rate is higher among apparently sporadic cases. This fact prevents the identification of individuals at the risk of heart failure that can lead to heart transplantation or sudden death. The identification of genes responsible for HCM has mainly relied on linkage analysis in large pedigrees [3] . However, this approach is not suitable for the study of more common smaller pedigrees due to the lack of statistical power. The recent development of next-generation sequencing methods represents a powerful and unbiased strategy to uncover the genetic changes that are responsible for hereditary diseases [5] , [6] , [7] . Here we perform exome-capture followed by next-generation sequencing to identify the putative genetic alterations present in one family with HCM that lacked mutations in known genes involved in this disease. On the basis of these studies, together with additional genome sequencing analysis of 92 subjects with HCM, we suggest that mutations in the FLNC gene encoding the sarcomeric protein filamin C are a novel cause of HCM. Study subjects A 53-year-old woman (patient CAR2_III-1) was diagnosed with HCM at 20 years of age on the basis of published criteria, including electrocardiography showing left ventricular hypertrophy and echocardiography showing a hypertrophic septum (27 mm) [8] , [9] . She was treated with beta-blockers, but 12 years later developed atrial fibrillation and received an electrical cardioversion and was treated with amiodarone. After a second failed cardioversion, magnetic resonance with late gadolinium enhancement showed extensive areas of fibrosis affecting the septum, apex and anterior wall. She received an implantable cardioverter defibrillator (ICD), without discharges to date. Currently, she is under treatment with beta-blockers, in NYHA grade I and with a left-ventricular outflow obstruction (LVOTO) of 30 mm Hg. The case is consistent with familial HCM based on the presence of additional members of the family with HCM. The pedigree of this family and the main characteristics of the affected members are shown in Fig. 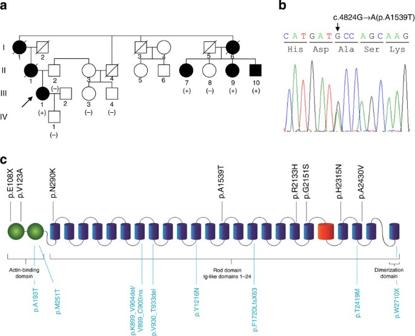Figure 1: Familial hypertrophic cardiomyopathy due to mutations inFLNC. (a) Pedigree of the affected family (CAR2). Solid symbols indicate affected subjects, and open symbols unaffected relatives. Squares denote male family members, circles female members and slashed deceased members. Arrow indicates index case. (b) Partial sequence electropherogram of theFLNCgene with the nucleotide substitution identified in the three affected members analysed (family members III-1, II-7 and II-9). The heterozygous mutation c.4824G>A (arrow) causes a missense substitution p.A1539T. (c) Schematic representation of the filamin C protein with the position of the eight mutations identified in this work in patients with HCM (up) as well as the mutations reported in patients with myofibrillar myopathy (down). 1 and Supplementary Table 1 , respectively. Thus, her mother suffered sudden death during labor at 34 years of age, and her grandmother and grand-aunt died at the age of 62 and 55, respectively, from cardiac causes. Two additional relatives (CAR2_II-7 and CAR2_II-9) ( Fig. 1 ) were diagnosed with HCM at 45 and 82 years of age. Nucleotide-sequencing analysis of all coding exons plus intronic flanking regions of sarcomeric genes previously associated with HCM, including MYH7 , MYBPC3 , TNNT2 , TNNI3 , TPM1 , ACTC1 , TNNC1 , MYL 2 and MYL3 , failed to show any mutation in this patient. Figure 1: Familial hypertrophic cardiomyopathy due to mutations in FLNC . ( a ) Pedigree of the affected family (CAR2). Solid symbols indicate affected subjects, and open symbols unaffected relatives. Squares denote male family members, circles female members and slashed deceased members. Arrow indicates index case. ( b ) Partial sequence electropherogram of the FLNC gene with the nucleotide substitution identified in the three affected members analysed (family members III-1, II-7 and II-9). The heterozygous mutation c.4824G>A (arrow) causes a missense substitution p.A1539T. ( c ) Schematic representation of the filamin C protein with the position of the eight mutations identified in this work in patients with HCM (up) as well as the mutations reported in patients with myofibrillar myopathy (down). Full size image Exome sequencing of a patient with familial HCM Exome sequencing was performed on patient CAR2_III-1 ( Fig. 1 ). More than 80% of the exome regions were callable and 19,467 variants were identified. We confirmed that no mutations in genes previously associated with HCM were present in this patient. After removing common polymorphisms, a total of 128 variants potentially affecting protein function due to the introduction of missense, nonsense, splicing or frameshifts in the coding regions were identified in this patient ( Supplementary Table 1 ). From these gene variants, we searched for those predicted to affect the function of the protein and presenting cardiac-specific expression, with the finding that FLNC —encoding the muscle-specific filamin C and implicated in myocyte differentiation—had a missense mutation in this patient (p.A1539T). This filamin is localized at the Z-discs of the sarcomere and interacts with other sarcomeric proteins, including myozenin-2 and myotilin [10] , [11] . To further evaluate the possibility that FLNC could be a novel gene associated with familial HCM, we next analysed whether the FLNC variant identified in this patient segregated with the disease in this family. Analysis of nine available members of this pedigree (four affected and five non-affected) ( Fig. 1 ) revealed that the identified variant (p.A1539T) segregated with the disease. Three additional members of the family (I-1, II-1 and I-6), who were obligate carriers of the FLNC p.A1539T variant but for which DNA was not available for analysis, died due to cardiac failure and were considered affected for the purpose of this analysis. Individual II-4, deceased at the age of 90, did not show symptoms of HCM, had normal electrocardiograms and was considered non-affected, although lack of DNA from this individual prevented genotyping. Inclusion of those obligate carriers in the analysis resulted in evidence of linkage between the FLNC variant p.A1539T and HCM in this family (LOD score=2.33). FLNC variants in families with HCM To examine whether FLNC variants could be also present in other families with HCM, we performed nucleotide-sequencing analysis of the 48 FLNC coding exons in an additional set of 92 HCM cases (19% with familial HCM and 81% apparently sporadic) who were negative for mutations in the aforementioned sarcomeric genes, using pooled-PCRs followed by next-generation sequencing. This study revealed six additional unique missense variants and a nonsense variant ( Fig. 1 and Table 1 ). Overall, we identified eight unique variants in a total of nine subjects with HCM. 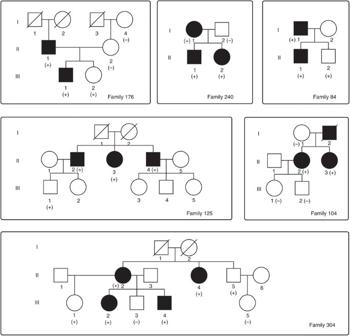Figure 2: Pedigrees of families with mutations inFLNC. Solid symbols indicate affected subjects, and open symbols unaffected relatives.FLNCmutation carriers are denoted with a ‘+’ symbol, and noncarriers with a ‘−’ symbol. Sequencing of available family members resulted in the finding of 18 additional subjects carrying the identified FLNC variants in the index cases ( Supplementary Table 2 ). None of these FLNC variants were present in >400 subjects of the Spanish population, 1000genomes or the exome-sequencing project (ESP), with the exception of variant p.A2430V, for which 2 alleles, out of 12,624 analysed, were identified in the ESP. Variant FLNC p.A2430V is the only one classified as neutral by the SIFT prediction server, and therefore this variant might constitute a rare polymorphism in the FLNC gene, although the presence of individuals with HCM on the ESP project cannot be ruled out. To determine whether the number of patients with FLNC mutations observed in our sample was different from that expected in the general population, we compared these results with those of the ESP project for the European–American population. We found 98 out of 4,200 individuals from the ESP project with variants predicted as deleterious by SIFT and PolyPhen, including some frameshifts and stop codons in the C-terminal region similar to those described for myofibrillar myopathy [12] . By contrast, we had seven patients out of 92 with FLNC variants predicted as deleterious by both algorithms (Fisher’s Exact Test P =0.0068, OR=3.44, 95% CI: 1.31–7.68), indicating that is unlikely to obtain this distribution of mutations by chance. In addition, we observed strong cosegregation of FLNC variants and clinical status among eight families affected by HCM ( Fig. 2 and Supplementary Table 2 ) (combined LINKAGE LOD score=4.1). Among the 16 individuals carrying a FLNC variant who were older than 40, and for whom data were available, 14 had HCM symptoms, resulting in a penetrance >87%. 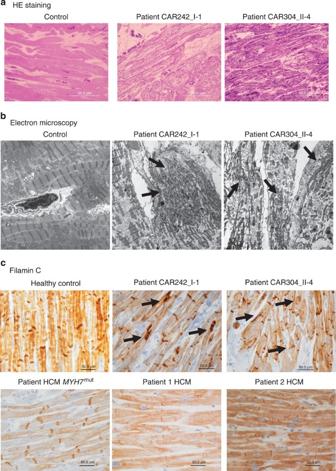Figure 3: Consequences ofFLNCmutations in cardiac tissue of HCM patients. (a) H&E staining of heart explants from two transplanted cases shows sarcomere disarray and aggregates of sarcomeric structures not present in the heart of a healthy control subject. (b) Ultrastructural analysis of cardiac tissue from the same subjects. Myofibre disarray, sarcomere disorganization and presence of deposits are visible in the cardiac tissue of HCM patients, but not in the control (magnification × 5,000). (c) Immunohistochemical staining reveals the presence of filamin C in the protein aggregates (arrows) occurring in cardiomyocytes of patients withFLNCmutations. Analysis of heart samples from a healthy control as well as three HCM patients, one caused by a mutation inMYH7, and two without mutations in sarcomeric genes orFLNC, revealed large nuclei and larger fibre diameter, but not filamin C aggregates. No differences in incidence between males and females, age at diagnosis, left ventricular obstruction tract outflow or the presence of cardiac symptoms were observed between subjects with or without variants in FLNC ( Supplementary Table 3 ). Septums appeared to be thinner in FLNC mutation carriers with hypertrophy ( n =20; 16 versus 19.2 mm, P <0.05), and the presence of FLNC mutations was associated with a higher frequency of familial history of HCM (55 versus 17.8%, P <0.01). Two patients underwent heart transplantation due to cardiac insufficiency secondary to diastolic failure, and both carried mutations in FLNC (cases CAR242_I-1 and CAR304_II-4). Interestingly, five of the nine families with mutations in FLNC had cases of sudden cardiac death (4 early, 1 late), in comparison with 23 (10 early, 13 late) out of 84 cases without variants in FLNC (56 versus 27%, P <0.05). Table 1 FLNC mutations identified in families with hereditary cardiomyopathy. Full size table Figure 2: Pedigrees of families with mutations in FLNC . Solid symbols indicate affected subjects, and open symbols unaffected relatives. FLNC mutation carriers are denoted with a ‘+’ symbol, and noncarriers with a ‘−’ symbol. Full size image FLNC variants affect cardiac muscle structure Interestingly, mutations in FLNC have been previously associated with myofibrillar myopathy (MIM 609524) [12] , [13] . However, none of the patients diagnosed with HCM in our study showed symptoms of myofibrillar myopathy, including nine subjects older than 44 years, which is the mean age at onset reported for the most common mutation in FLNC (p.W2710X) [13] . Four HCM patients with mutations in FLNC were studied by electromyography and magnetic resonance imaging with negative results. Histological analysis of skeletal muscle biopsies from two patients with HCM and FLNC variants (p.A1539T, case CAR2_III-1, and p.H2315N, case CAR125_II-2) showed intact sarcomeric structures, normal ATPase, SDH and NADH staining, as well as the absence of small aggregates, which are characteristic of myofibrillar myopathy ( Supplementary Fig. 1 ). The FLNC mRNA expression level in a skeletal muscle biopsy was similar to that found in individuals without FLNC mutations ( Supplementary Fig. 2 ). In addition, no evidence of filamin C or desmin aggregates, spheroid bodies or deposits, features typically found in skeletal muscles from subjects with myofibrillar myopathy and FLNC mutations [12] , [14] , [15] were observed in our HCM patients ( Supplementary Figs 1 and 2 ). Histological analysis of cardiac muscle sections from two transplanted subjects with FLNC mutations (p.G2151S, case CAR242_I-1 and p.A1539T, case CAR304_II-4) revealed marked sarcomeric abnormalities, including myofibrillar disarray, sarcomeric aggregates and fibrosis not observed in control hearts from either three HCM patients without mutations in FLNC or from a healthy subject ( Fig. 3 and Supplementary Fig. 3 ). Electron microscopy examination showed strong Z-band irregularities and myofibrillar disarray, as well as rod formation in cardiomyocytes from these patients. Immunohistochemical staining confirmed the presence of filamin C in the sarcomeric aggregates observed in cardiac myocytes from patients with FLNC mutations ( Fig. 3 and Supplementary Fig. 3 ). Finally, and similar to subjects with myofibrillar myopathy, we found that 34% (9/26) of the subjects with HCM and mutations in FLNC had elevated levels of serum creatine kinase, in contrast to 6% (5/82) of patients with HCM and lacking FLNC variants ( P <10 −4 ) ( Supplementary Table 2 ). Serum creatine kinase levels varied from normal to up to sixfold of the upper normal limit. All nine subjects with elevated serum creatine kinase levels belonged to three of the seven analysed families, and in these families all carriers of FLNC variants (p.V123A, p.H2315N and p.A2430V) showed high creatine kinase levels. Figure 3: Consequences of FLNC mutations in cardiac tissue of HCM patients. ( a ) H&E staining of heart explants from two transplanted cases shows sarcomere disarray and aggregates of sarcomeric structures not present in the heart of a healthy control subject. ( b ) Ultrastructural analysis of cardiac tissue from the same subjects. Myofibre disarray, sarcomere disorganization and presence of deposits are visible in the cardiac tissue of HCM patients, but not in the control (magnification × 5,000). ( c ) Immunohistochemical staining reveals the presence of filamin C in the protein aggregates ( arrows ) occurring in cardiomyocytes of patients with FLNC mutations. Analysis of heart samples from a healthy control as well as three HCM patients, one caused by a mutation in MYH7 , and two without mutations in sarcomeric genes or FLNC , revealed large nuclei and larger fibre diameter, but not filamin C aggregates. Full size image Functional analysis of FLNC mutations Notably, all the identified FLNC variants affected highly conserved residues in the protein encoded by this gene, from fish to human ( Supplementary Fig. 4 ). We also observed that FLNC variants were non-randomly distributed within filamin C ( Fig. 1 ), as they were mainly clustered on the N-terminal (actin-binding domain and first rod repeat) or C-terminal (last four rod repeats) portions of the protein. These data strongly suggest that FLNC variants found in subjects with HCM might impair the function of this sarcomeric protein. To evaluate this possibility, we generated four filamin C full-length cDNA clones containing the p.V123A, p.A1539T, p.R2133H or p.A2430V mutations identified in HCM patients. H9C2 rat cardiac myoblasts were nucleofected with wild-type FLNC or the mutant constructs, and the formation of insoluble filamin C aggregates was determined using sequential detergent extraction. Western blot analysis revealed that wild-type FLNC was exclusively present in the soluble fraction, while three of the four analysed mutants (p.V123A, p.R2133H and p.A2430V) could be detected in the insoluble fraction ( Fig. 4a ), consistent with the formation of protein aggregates when expressed in cardiac myoblasts. In addition, expression of two of the analysed mutants (p.A1539T and p.R2133H) also resulted in the formation of actin aggregates ( Fig. 4a ). 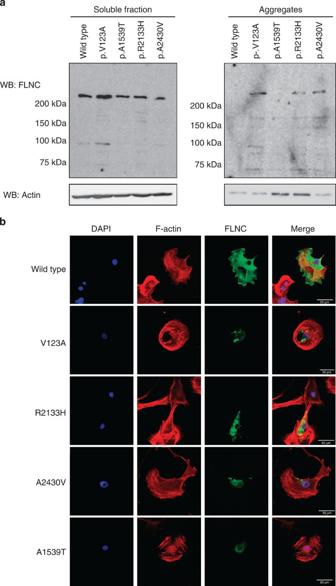Figure 4: Functional analysis ofFLNCmutants. (a) H9C2 rat cardiac myoblast cells were transiently transfected with expression vectors encoding DDK-tagged wild-typeFLNCor mutants p.V123A, p.A1539T, p.R2133H or p.A2430V. Soluble and insoluble protein extracts were subjected to SDS–PAGE, and filamin C or actin was detected by western blot using an anti-DDK or anti-actin antibodies, showing the presence of insoluble filamin C and actin when some mutants were expressed. (b) Subcellular distribution of ectopically expressed FLNC wild type and mutants in neonatal rat cardiac myocytes was analysed by immunofluorescence and confocal microscopy. Filamin C distribution was detected using an anti-DDK antibody, actin fibres were stained with phalloidin and nuclei were counterstained with DAPI. Ectopic expression of mutantFLNCconstructs resulted in the formation of perinuclear protein aggregates not observed in wild-typeFLNC. Figure 4: Functional analysis of FLNC mutants. ( a ) H9C2 rat cardiac myoblast cells were transiently transfected with expression vectors encoding DDK-tagged wild-type FLNC or mutants p.V123A, p.A1539T, p.R2133H or p.A2430V. Soluble and insoluble protein extracts were subjected to SDS–PAGE, and filamin C or actin was detected by western blot using an anti-DDK or anti-actin antibodies, showing the presence of insoluble filamin C and actin when some mutants were expressed. ( b ) Subcellular distribution of ectopically expressed FLNC wild type and mutants in neonatal rat cardiac myocytes was analysed by immunofluorescence and confocal microscopy. Filamin C distribution was detected using an anti-DDK antibody, actin fibres were stained with phalloidin and nuclei were counterstained with DAPI. Ectopic expression of mutant FLNC constructs resulted in the formation of perinuclear protein aggregates not observed in wild-type FLNC . Full size image Similarly, when these mutants were expressed in rat neonatal cardiac myocytes, we found that they form large filamin C aggregates as assessed by immunofluorescence and confocal microscopy ( Fig. 4b ). However, wild-type filamin C expression resulted in a cytoplasmic distribution, mainly associated with actin fibres, and absence of aggregate formation ( Fig. 4b ). We noticed some variability in the distribution pattern between different mutants. Interestingly, the p.V123A mutant, which by confocal microscopy showed the largest aggregates in rat cardiac myocytes, had also the strongest signal by western blot analysis in the insoluble fraction, thereby showing a close agreement between microscopic and biochemical methods, and supporting the formation of aggregates by these filamin C mutants. Overexpression of these mutants in C2C12 cell myotubes also resulted in the formation of protein aggregates, although they were smaller than those observed in cardiac myocytes ( Supplementary Figs 5 and 6 ). Together, these data support the hypothesis that the mutations in filamin C identified in HCM patients disrupt the structure of this sarcomeric protein, leading to the formation of protein aggregates that might finally impair sarcomere function. We describe here a family with an autosomal dominant HCM of unknown genetic basis. By means of whole-exome sequencing of the index case and subsequent target resequencing of a candidate gene in an additional set of 92 HCM patients, we have shown evidence of linkage between mutations in FLNC and familial HCM in eight independent families of Spanish origin. FLNC encodes the sarcomeric protein filamin C, a muscle-specific protein involved in myocyte differentiation and muscle function by interacting with proteins of both the Z-disc and the sarcolemma [16] . Mutations in genes encoding other sarcomeric proteins, including MYH7 , TPM1 , TNNT2 , MYL3 and TNNI3 , are responsible for a large fraction of HCM cases, indicating that the FLNC mutations identified in this work expand the number of sarcomeric genes implicated in this pathology. Mutations in FLNC had been previously shown to be responsible for myofibrillar myopathy [12] , [13] , [16] . However, none of our HCM patients showed symptoms of this filaminopathy, and none of the FLNC mutations identified in our study overlapped with those reported for myofibrillar myopathy. In fact, analysis of skeletal muscle biopsies from two HCM patients showed a normal muscle fibre histology and biochemistry, and lacked any of the myopathological or electrophysiological abnormalities described in myofibrillar myopathy patients. These findings, together with previous reports showing that different mutations within the filamin C molecule result in different myopathological features [16] , suggest that filaminopathies caused by FLNC mutations are not restricted to skeletal muscle disorders, but can generate a spectrum of muscle disorders with distinct involvement of skeletal and cardiac muscle abnormalities. This intriguing and interesting observation is not unprecedented. Thus, different mutations in the gene encoding the myosin heavy chain 7 ( MYH7 ) can result in either Laing-type early-onset distal myopathy [17] or HCM [3] , [18] , suggesting that mutations affecting different residues of these sarcomeric proteins can result in different clinical outcomes. Similarly, mutations in the lamin A/C gene ( LMNA ) can originate several different diseases including dilated cardiomyopathy 1A, Emery-Dreyfuss muscular dystrophy, lipodystrophy, mandibuloacral dysplasia, limb-girdle muscular dystrophy and Hutchinson-Gilford progeria syndrome. With the exception of Hutchinson-Gilford progeria, caused by de novo mutations affecting the C-terminal end of the protein, or lipodystrophy, caused by inherited mutations usually near the C-terminal end of the protein, all other pathologies are caused by LMNA mutations that are scattered along the length of the protein, and no genotype–phenotype segregation has been established [19] , [20] , [21] . Similarly, mutations in FHL1 , which usually cause skeletal muscle disease, have been shown to cause HCM with left ventricular diastolic dysfunction without skeletal muscle affection [22] , [23] . This situation is closely parallel to that of the FLNC mutations described in the present work, which are mainly clustered on the N- and C-terminal parts of the protein, but none of them overlap with previously described mutations causing myofibrillar myopathy [16] . Nevertheless, and taking into account that filamin C interacts with many proteins involved in muscle function, we can speculate that some mutations may have more impact in cardiac muscle or in skeletal muscle, depending on whether they affect specific domains or binding surfaces of this sarcomeric protein. In this regard, the finding that expression of these mutants in cardiac myocytes resulted in the formation of larger protein aggregates than when expressed in C2C12 myotubes supports a model in which interaction of these mutants with tissue-specific proteins, contributes to the predominant cardiac phenotype. In this regard, it is also remarkable that about one-third of myofibrillar myopathy patients with the most frequent mutation in FLNC (the German variant, p.W2710X) are reported to have cardiac abnormalities, although only two out of 25 patients had cardiomyopathy with left ventricular dysfunction [13] . These data suggest that the clinical spectrum of the different filaminopathies is highly dependent on the site of mutation within the filamin C molecule. In fact, and despite the absence of histological abnormalities or filamin C aggregates in skeletal muscle from our HCM patients, analysis of heart samples from two of them subjected to heart transplant due to their HCM revealed myofibrillar disarray and sarcomeric aggregates in cardiac muscle similar to those described in skeletal muscle of patients with myofibrillar myopathy. Furthermore, we have demonstrated that at least three of the mutations identified in HCM families disrupt the functional structure of the protein and lead to the formation of protein aggregates when expressed in cardiac myoblasts, further supporting a functional role for these mutations. In addition, expression of two of these mutants, including p.A1539T for which FLNC protein aggregates were not detected, resulted in the formation of actin aggregates. This suggests that expression of this mutant is also able to alter the cytoskeleton structure, raising the possibility that actin aggregation might contribute to HCM in some of these patients. Although loss of function mutations might contribute to the development of HCM in these patients, the fact that Flnc -deficient mice show a disruption of the skeletal muscle structure without apparent cardiac involvement [24] suggests that other mechanisms might be implicated in this process. Thus, the previous finding that Flnc -knockout mice are neonatally lethal, whereas heterozygous mice show no obvious phenotype, supports the hypothesis that the formation of protein aggregates, and not the lack of function of FLNC mutants, is responsible for the muscle alterations observed in these pathologies. In this regard, the fact that three out of the four mutants analysed in this study form protein aggregates when overexpressed in rat cardiac myocytes supports this hypothesis. Nevertheless, we cannot rule out that other molecular mechanisms might also contribute to the aetiology of the disease and might explain the fact that one of the four analyzed mutations (p.A1539T) did not form protein aggregates in our in vitro experimental system. In addition, and despite the apparent absence of a cardiac phenotype in mice lacking the last eight exons of Flnc , the medaka mutant zacro , which results from a homozygous nonsense mutation in the 15th rod domain of filamin C [25] , shows an enlarged heart and progressive skeletal muscle degeneration, thus reinforcing our proposal that this protein is central for cardiac function. Notably, we found a higher proportion of sudden cardiac deaths among families with FLNC mutations when compared with cases without FLNC mutations, thus providing an additional clinical dimension to the identification of high-risk patients carrying these mutations. In this regard, we observed that among the two families with the same FLNC mutation (p.A1539T), there were three cases of sudden death and one patient was transplanted, suggesting that this particular amino-acid change might have a greater impact on the clinical evolution of the disease. The presence of two asymptomatic carriers within these families (ages 12 and 52) allows a closer monitoring of these individuals to identify potential symptoms of HCM. Thus, echocardiographic follow-up of individual CAR304_II-5 (age 52) revealed an incipient hypertrophic septum (11 mm), compatible with an initial phase of HCM development. These results underscore the utility of these findings for the early detection of at risk individuals who can also benefit for specific treatment. Finally, we realize that the relatively small size of some of the families used in this study constitutes a limitation to achieve statistical significance by relaying only in sequencing data. In this regard, and in agreement with the guidelines for investigating causality of sequence variants in human disease [26] , we have combined sequencing information with expression data in the heart, statistical analysis of population-based variants in FLNC , as well as performed extensive functional validation of the identified mutations, which support the role of FLNC mutations in familial HCM. Nevertheless, future studies aimed at expanding the number of HCM families will be necessary to define the precise role of FLNC in HCM. In conclusion, by using exome-capture and next-generation sequencing we have identified FLNC as a potential new gene implicated in HMC, thereby demonstrating the utility of these approaches for the rapid and efficient identification of the genetic causes of inherited diseases. This work also underscores the relevance of filamins in cardiac pathologies and provides new insights for the appropriate molecular diagnosis and clinical management of carriers of FLNC mutations in HCM families. Study subjects All participants had provided written informed consent approved by the Ethics Review Board of the Hospital Universitario Central de Asturias (Oviedo, Spain). Peripheral blood leukocytes were collected and used for isolation of genomic DNA. Study subjects included a proband with a family history of HCM, as well as other members of her family ( Supplementary Table 2 , and Fig. 1 ). A panel of 92 additional patients with the same clinical characteristics and lacking mutations in known sarcomeric genes were also studied ( Supplementary Table 3 ). Exome sequencing Genomic DNA was extracted from peripheral blood leukocytes with a Qiagen kit according to the manufacturer’s instructions (Qiagen, Germany). Exome capture from patient CAR_III-1 genomic DNA was performed using a SureSelectXT Human All Exon 50 Mb Kit (Agilent). In brief, 3 μg of genomic DNA was sheared with a Covaris S2 instrument and used for the construction of a paired-end sequencing library as described in the paired-end sequencing sample preparation protocol provided by Illumina [27] . Enrichment of exonic sequences was then performed using the Sure Select Human All Exon 50 Mb Kit (Agilent Technologies) following the manufacturer’s instructions. Exon-enriched DNA was pulled down by magnetic beads coated with streptavidin (Invitrogen), followed by washing, elution and 18 additional cycles of amplification of the captured library. The enriched library was sequenced (2 × 76 bp) using a HiSeq 2000 instrument (Illumina). Exome sequence data analysis Sequence data were analysed using a custom pipeline as previously described [5] . In brief, reads were mapped to the human reference genome (GRCh37) using BWA [28] with the sampe option, and a BAM file was generated using SAMtools [29] . Optical or PCR duplicates were removed using Picard ( http://picard.sourceforge.net/index.shtml ). Bases were initially called using SAMtools and BCFtools. Variants present in dbSNP135 with a minor allele frequency >0.01, or present in >2% of individuals of Spanish origin without previous history of HCM for which exome data were available as part of the CLL-ICGC project [30] , were discarded as common polymorphisms. Variants potentially affecting protein function, including non-synonymous variants, frameshifts in the coding sequence, or variants potentially affecting splicing, were analysed. Clinical validation sequencing For the validation studies, the exonic regions of FLNC were amplified and sequenced in a validation series of 92 patients with HCM using specific primers and SMIPS [31] , a pooled-sequencing approach combined with next-generation sequencing ( Supplementary Table 4 ). Data analysis was performed using custom scripts to identify variants in the pooled sequence data, and mutations were confirmed in additional subjects from the same families using Sanger sequencing. For the calculation of LOD scores, parametric linkage was performed using the program LINKAGE [32] . Only family members for which genotype was available were considered for the analysis, and other members were scored as unknown, with the exception of individuals I-1, II-1 and I-6 from family 2, who were affected and obligate carriers but for whom no DNA was available, and were considered affected carriers. Skeletal muscle studies To evaluate skeletal muscle affection, HCM patients were studied by electromyography and/or magnetic resonance. In addition, tru-cut muscular biopsies were performed to patients CAR2_III-1 and CAR125_II-1. Both signed an informed consent for the use of samples in research, according to the national regulations of LIB 14/2007. Samples were obtained from the right quadriceps through a small (2 mm) skin incision and a tru-cut biopsy needle (Care Fusion 14G 7.6 cm). The skin and subcutaneous tissue down to the muscle sheet were previously infiltrated with 2% Mepivacaine (Braun). A small sample was immediately fixed in glutaraldehyde, at room temperature. In addition, a small piece was fixed in 5% formalin and paraffin embedded. The remaining of the muscular sample was observed under the stereoscopic microscope. Using a thin gauge, fibres were oriented transversally and snap-frozen on liquid nitrogen-freezing isopentane. Thin 3-μm sections were obtained with a cryostat and stored at −80 °C before use. Histochemistry Histochemical techniques were performed according to the literature [33] for Engel-Gomori trichrome, succinate dehydrogenase (SDH), NADH dehydrogenase (NADH), cytochrome C oxidase (COX), esterase and adenosine triphosphatase (ATPase) pH 9.4. Immunohistochemistry Immunohistochemistry was performed on paraffin 3-μm thick sections, previously heated at 60 °C, then cleared and dehydrated in xylene and graded alcohols. Antigen retrieval was performed by heating in with a Tris Borate EDTA buffer (pH 8.4). Endogen peroxidase activity was quenched by incubation in TBS-T containing 3% hydrogen peroxide. Each incubation step was carried out at room temperature and followed by three sequential washes in TBS-T. To block non-specific binding, tissues were incubated for 20 min in TBS-T containing 10% bovine serum albumin (BSA). Samples were incubated with a primary rabbit polyclonal antibody against filamin C (Novus Biologicals, Littleton, CO) at 1:25 dilution, followed by incubations with a biotinylated OMNImap secondary antibody for 15 min, peroxidase-labelled streptavidin and diaminobenzidine substrate. Control immunohistochemical staining was performed following the same procedure but omitting the primary antibody. Procedures were performed in a Discovery Ventana system (Roche). Slides were dehydrated and mounted with a xylene-based medium. Electron microscopy Muscle samples were fixed in glutaraldehyde for 3 h, and post-fixed in osmic tetroxide and embedded in Epon resin (Embed-812) using an automated tissue processor (Reichert Lynx). Ultrathin sections were prepared with a diamond knife using an ultramicrotome (Ultracut Reigert-Jung), and post stained with uranyl acetate and lead citrate. The ultrastructural observations were performed using a Jeol 1200 electron microscope equipped with a digital camera. Heart samples Heart samples from transplant receptors CAR242_I-1 and CAR304_II-4 were studied in parallel with control hearts from a healthy donor and three HCM patients without mutations in FLNC , one of them with a mutation in the sarcomeric gene MYH7 , and two others without mutations in known genes. Coronary sections were performed following 5% formaldehyde fixation. Representative samples of right and left ventricles, septal area and coronaries were paraffin embedded. Serial 3-μm sections were obtained for H&E staining. Additional sections were used for immunohistochemistry. The procedure was the same as for the peripheral muscle with a control sample placed on the same slide for each case. For ultrastructural studies, small (2 mm) left ventricle samples were obtained from paraffin blocks using a razor blade. Samples were deparaffinized and prepared for ultrastructural studies following the same procedure as the peripheral muscle biopsies. Directed mutagenesis of full-length filamin C A full-length cDNA clone for filamin C (NM_001458) with an N-terminal Myc-DDK-Tag was obtained from OriGene (Rockville, MD). Site-directed mutagenesis was performed to generate four clones with the p.A1539T, p.V123A, p.R2133H and p.A2430V mutations, respectively, using a QuikChange II XL Site-Directed Mutagenesis kit according to the manufacturer’s recommendations (Stratagene) and specific oligonucleotides ( Supplementary Table 5 ). Introduction of the correct mutation and absence of additional mutations was verified by Sanger sequencing. Cell culture and immunofluorescence Rat cardiac myoblast cell line H9C2 was kindly provided by Dr M. Mittelbrunn. Cells were grown in DMEM supplemented with 10% new born calf serum and L -Glutamine. Cells were transfected using Amaxa SF cell line 4D-Nucleofector X Kit by Lonza following the manufacturer’s instructions. In brief, 3 × 10 6 cells were nucleofected with 2 μg of each plasmid and 48 h after transfection the presence of protein aggregates was analysed by sequential detergent extraction of proteins. Neonatal Rat Cardiac Myocytes were obtained by Lonza. Cells were grown in rCMC Medium, containing Basal Media (RCBM Medium) supplemented with Horse serum, Fetal Bovine Serum, Gentamicin/Amphotericin-B and Bromo-2′-deoxyuridine (BrdU) according to the manufacturer’s instructions. Cells were transfected using the Amaxa rat Cardiomyocyte Neo Nucleofector Kit by Lonza. In brief, 1 × 10 6 cells were nucleofected with 2 μg of each plasmid and 48 h after transfection cells were analysed by immunofluorescence. Basically, cells were washed with PBS, fixed with 4% (v/v) formaldehyde and permeabilized by incubation with 0.2% Triton X-100 in PBS. Cells were washed, blocked with 10% normal goat serum in PBS, followed by incubation using an anti-DYKDDDDK Tag Antibody (Cell Signaling) diluted in 1% FCS in PBS. Following multiple washes, cells were incubated with an Alexa Fluor 488-conjugated goat anti-rabbit IgG antibody (1:500) and with Phalloidin-Alexa 568 (Molecular Probes) for 1 h at room temperature. Nuclei were stained with 4′,6-diamidino-2-phenylindole (DAPI), coverslips were mounted on slides and cells imaged with a Leica SP2 confocal microscope (Leica Microsystems). C2C12 myoblasts were grown on Dulbecco’s modified Eagle’s medium (DMEM, Gibco) containing 4 mM L -glutamine (Gibco) and 10% fetal calf serum (Gibco), and sodium pyruvate. To express wild-type and mutant filamin C, cells were transiently transfected with 1 μg of the appropriate plasmid using Lipofectamine (Invitrogen), grown for 24 h and then placed on glass coverslips. To induce myotube formation, cells were switched to medium containing 5% horse serum, cultured for 72 h and analysed by immunofluorescence as above. Sequential detergent extraction of proteins and western blot For protein extraction, cultured cells were washed twice with 1 × PBS and resuspended in TEN buffer (10 mM TrisHCl pH 8.0, 1 mM EDTA, 100 mM NaCl, 50 mM iodoacetamide) supplemented with complete protease inhibitor cocktail without EDTA (Roche) and 0.5% NP-40. Cell lysates were centrifuged at 13,000 g for 5 min, and supernatant was conserved as soluble fraction. The insoluble fraction was further solubilized using TEN buffer containing 2% SDS, sonicated and centrifuged at 16,000 g for 10 min. This latter supernatant was conserved as the insoluble fraction. Protein concentration was evaluated with the bicinchoninic acid technique (Pierce BCA protein assay kit). Proteins were run in SDS-PAGE gels, transferred to nitrocellulose membranes, blocked with 5% non-fat dry milk in TBS-T buffer (20 mM Tris pH 7.4, 150 mM NaCl, 0.05% Tween 20) and incubated overnight at 4 °C with the following primary antibodies: anti-DDK tag antibody (Cell Signaling) and anti-actin (Sigma). Primary antibodies were detected with horseradish peroxidase-conjugated species-specific secondary antibodies (Jackson Immunoresearch or Thermo Scientific) with Luminata Forte Western HRP Substrate (Millipore) using a LAS-300 FUJIFILM. How to cite this article: Valdés-Mas, R. et al . Mutations in filamin C cause a new form of familial hypertrophic cardiomyopathy. Nat. Commun. 5:5326 doi: 10.1038/ncomms6326 (2014). Accession codes: Whole-exome sequence data for patients with HCM have been deposited in the European Genome-phenome Archive (EGA) under the accession code EGAS00001000970.